Edge-terminated molybdenum disulfide with a 9.4-Å interlayer spacing for electrochemical hydrogen production Layered molybdenum disulfide has demonstrated great promise as a low-cost alternative to platinum-based catalysts for electrochemical hydrogen production from water. Research effort on this material has focused mainly on synthesizing highly nanostructured molybdenum disulfide that allows the exposure of a large fraction of active edge sites. Here we report a promising microwave-assisted strategy for the synthesis of narrow molybdenum disulfide nanosheets with edge-terminated structure and a significantly expanded interlayer spacing, which exhibit striking kinetic metrics with onset potential of −103 mV, Tafel slope of 49 mV per decade and exchange current density of 9.62 × 10 −3 mA cm −2 , performing among the best of current molybdenum disulfide catalysts. Besides benefits from the edge-terminated structure, the expanded interlayer distance with modified electronic structure is also responsible for the observed catalytic improvement, which suggests a potential way to design newly advanced molybdenum disulfide catalysts through modulating the interlayer distance. The blueprint of ‘hydrogen (H 2 ) economy’ is to store energy from renewable sources, such as sunlight or wind, into the chemical bond of H 2 via electrolysis of water, which then can be released through the reverse reaction in fuel cells on demand [1] . However, the scalable production of H 2 from water significantly depends on the efficiency of electrocatalytic materials. Ideal electrocatalysts must be, stable and capable of reducing water rapidly at potentials close to its thermodynamic value (2H + +2e − →H 2 ; 0−0.059 × pH, V versus normal H 2 electorde at 298 K) [2] , [3] . Although platinum (Pt) and its alloys can catalyse H 2 evolution reaction (HER) at potentials slightly below the thermodynamic potential for the H + /H 2 couple [2] , [3] , [4] , the high cost and scarcity of Pt pose tremendous limitation to widespread adoption. Therefore, the critical determinant of the energy storage in electrolytic systems is to develop robust and efficient alternative catalysts that are cheap and Earth abundant. Remarkable advances have been made recently regarding the use of chalcogenides of cobalt [5] , [6] , [7] , [8] , [9] , nickel [8] , [10] , molybdenum [9] , [11] , [12] , [13] , [14] , [15] , [16] , [17] , [18] , [19] and tungsten [15] , [20] , [21] as promising noble metal-free catalysts for HER. Among these materials, molybdenum disulfide (MoS 2 ), a widely used industrial catalyst for hydrodesulfurization of petroleum [22] , has received special attention and the catalytic active sites were identified theoretically [23] and experimentally [24] . Similar to many inorganic solids, the HER activity of MoS 2 is localized to the rare edge surfaces, whereas the (0001) basal planes are relatively inactive [23] , [24] , [25] . Motivated by this understanding, intense research efforts have been focused on developing highly nanostructured MoS 2 to maximize the number of exposed edge sites, including crystalline [26] , [27] , [28] , [29] and amorphous materials [12] , [15] , [30] , [31] , metallic 1T polymorph [9] , [32] , vertically aligned structures [33] , [34] and molecular mimics [25] . Other strategies to improve HER performance include incorporating MoS 2 with conductive materials by taking advantage of synergetic coupling effects [34] , [35] , [36] , [37] , [38] or doping first-row transition metal ions (for example, Fe, Co and Ni) into MoS 2 to optimize its catalytic sites at S-edges [26] , [39] . Despite striking achievements, many practical challenges still remain to improve the activity and stability of MoS 2 -based catalysts. Here, we report a class of colloidal MoS 2 nanostructure with edge-terminated and interlayer-expanded (ET&IE) features that exhibits high activity and stability towards HER in acidic water. Its fast kinetic metrics (including onset potential of −103 mV and the Tafel slope of 49 mV per decade) demonstrate superior electrocatalytic activity relative to the reported MoS 2 -only catalysts. In addition to the benefit of edge-terminated structure, the expansion of interlayers can further modify electronic structures and electrical conductivity of MoS 2 edge sites, leading to improved performance. This study hints at the promise of cheap and efficient HER electrocatalysts by modulating interlayer distance in two-dimensional atomic-layered materials. Microwave-assisted synthesis of ET&IE MoS 2 The ET&IE MoS 2 were synthesized through reduction of (NH 4 ) 2 MoS 4 in N , N -dimethylformamide (DMF) with the assistance of microwave heating. Compared with conventional heating methods, microwave-assisted synthesis is a greener strategy with high-level thermal management and dramatically reduced reaction time and therefore new nanostructured materials are likely to be achieved [40] . Reaction at 240 °C for 2 h results in a yield of ∼ 93% of ET&IE MoS 2 , demonstrating the rapid and efficient microwave chemistry. A schematic overview of the synthesis procedure is shown in Fig. 1 and the details are described in the Methods. The morphology and microstructure of MoS 2 prepared at different temperatures was studied by transmission electron microscopy (TEM) ( Fig. 2a–c ) and high-resolution TEM (HRTEM) ( Fig. 2d–f ). Reaction at low temperature (for example, 190 °C) forms reticulated network of amorphous materials ( Fig. 2a ), where some tiny MoS 2 -layered crystals appear ( Fig. 2d ), indicating the formation of crystalline nuclei from the amorphous matrix. Increasing reaction temperature results in the formation and growth of crystalline nuclei into larger MoS 2 nanocrystals via consumption of the amorphous materials. For example, MoS 2 synthesized at 240 °C exhibits a sheet-like morphology with sizes of tens of nanometres ( Fig. 2b ). HRTEM image in Fig. 2e clearly shows the resolved S–Mo–S layers with a curved stripe-like feature ( Supplementary Fig. 1 ) and the layer-to-layer spacing is about 9.4 Å. Further increasing temperature to 260 °C produces three-dimensional flower-like MoS 2 with better crystallinity ( Fig. 2c and inset). HRTEM image of a typical MoS 2 flower reveals that it is built from interlaced crystalline MoS 2 nanosheets ( Fig. 2f ). 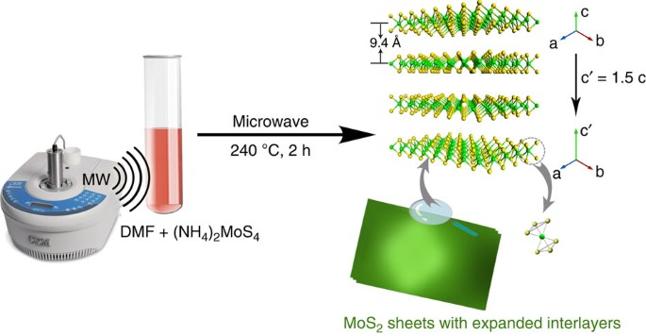Figure 1: Schematic illustration of the synthesis of ET&IE MoS2. Thecaxis of the as-synthesized MoS2shows about 1.5 × expansion as compared with that of standard 2H–MoS2phase. Green and yellow balls indicate Mo and S atoms, respectively. Figure 1: Schematic illustration of the synthesis of ET&IE MoS 2 . The c axis of the as-synthesized MoS 2 shows about 1.5 × expansion as compared with that of standard 2H–MoS 2 phase. Green and yellow balls indicate Mo and S atoms, respectively. 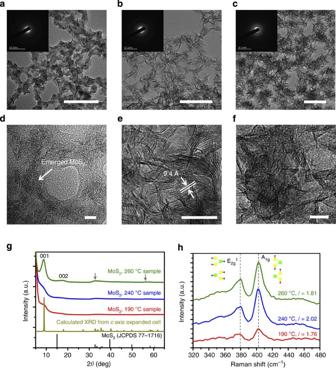Figure 2: Characterization of the MoS2nanosheets. (a–c) TEM images of MoS2nanostructures synthesized at 190 °C (a), 240 °C (b) and 260 °C (c). Scale bars, 100 nm. The insets in (a–c) show corresponding SAED patterns, respectively. (d–f) HRTEM images of MoS2nanostructures synthesized at 190 °C (d), 240 °C (e) and 260 °C (f). Scale bars, 10 nm. (g) X-ray diffraction patterns of MoS2nanostructures synthesized at different temperatures. The calculated pattern fromcaxis expanded MoS2cell and the standard pattern of the pristine 2H–MoS2(JCPDS 77-1,716) are shown as reference. (h) Raman spectra of the different MoS2products. The larger relative intensity ofA1g/E2g1for 240 °C sample (I=2.02) suggests its edge-terminated structure. Full size image Figure 2: Characterization of the MoS 2 nanosheets. ( a – c ) TEM images of MoS 2 nanostructures synthesized at 190 °C ( a ), 240 °C ( b ) and 260 °C ( c ). Scale bars, 100 nm. The insets in ( a – c ) show corresponding SAED patterns, respectively. ( d – f ) HRTEM images of MoS 2 nanostructures synthesized at 190 °C ( d ), 240 °C ( e ) and 260 °C ( f ). Scale bars, 10 nm. ( g ) X-ray diffraction patterns of MoS 2 nanostructures synthesized at different temperatures. The calculated pattern from c axis expanded MoS 2 cell and the standard pattern of the pristine 2H–MoS 2 (JCPDS 77-1,716) are shown as reference. ( h ) Raman spectra of the different MoS 2 products. The larger relative intensity of A 1g / E 2g 1 for 240 °C sample ( I =2.02) suggests its edge-terminated structure. Full size image Figure 2g presents the X-ray diffraction patterns of these samples, which are significantly different from that of bulk 2H–MoS 2 (JCPDS 77-1,716; Supplementary Fig. 2 ). Two new peaks with diploid relationship appears at low-angle region correspond to (001) and (002) reflections with d spacings of 9.4 and 4.7 Å, respectively. In comparison to the d spacing of 6.15 Å for pristine 2H–MoS 2 , the expanded interlayers of our samples is likely due to the intercalation of oxidized DMF species into two S–Mo–S layers ( Supplementary Fig. 3 ). The asymmetric nature of the reflection at 2 θ ≈32.7° revealed the presence of stacking faults [41] among MoS 2 layers as a result of a – b plane gliding caused by intercalated DMF species. A recent work also reported a large interlayer spacing of 9.5 Å in hydrothermally prepared MoS 2 , which however was ascribed to oxygen incorporation [29] . Unlike the product formed at 260 °C, the barely recognizable diffraction peaks of other two samples indicate the low crystallinity, which is consistent with their selected-area electron diffraction (SAED) patterns. Particularly, the greatly broad first peak for 240 °C sample was the result of its curly and crossed edge-terminated structure ( Fig. 2e ). The calculated X-ray diffraction pattern using an interlayer spacing of 9.4 Å along the c axis was found to agree well with experimentally collected patterns ( Fig. 2g ). Energy-dispersive X-ray spectra showed that the as-synthesized samples are mainly composed of Mo and S ( Supplementary Fig. 4 ). Raman spectra in Fig. 2h exhibited two distinct peaks at 379.2 cm −1 and 402.7 cm −1 , which correspond to the in-plane Mo–S phonon mode ( E 2g 1 ) and the out-of-plane Mo–S mode ( A 1g ) of typical MoS 2 -layered structure, respectively [33] , [37] . The relative intensities of A 1g / E 2g 1 provide texture information on the surface of deposited MoS 2 films and the largest ratio of 2.02 for 240 °C sample suggests that it favours the vibration of A 1g mode and thus the best edge-terminated structure [33] , [37] , which is consistent with the TEM observations ( Fig. 2a–f ). The phase and morphology evolutions of ET&IE MoS 2 were also studied by time-dependent reactions at 240 °C and the results are presented in Supplementary Figs 5 and 6 . Electrocatalytic HER activity The electrocatalytic properties of ET&IE MoS 2 for evolving H 2 were evaluated in Ar-saturated 0.5 M H 2 SO 4 electrolyte and compared with state-of-the-art Pt/C catalyst. The ohmic potential drop (iR) losses from the solution resistance were corrected. The electrodes were kept rotating at 1,600 r.p.m throughout the measurements in order to remove in situ produced H 2 bubbles. 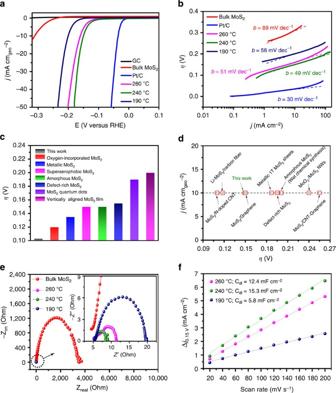Figure 3: Electrocatalytic hydrogen evolution of the catalysts. (a) Polarization curves for HER on bare glassy carbon electrode and modified glassy carbon electrodes comprising MoS2nanosheets synthesized from different temperatures, bulk MoS2and a high quality commercial Pt/C catalyst. Catalyst loading is 0.28 mg cm−2for all samples. Sweep rate: 5 mV s−1. (b) Tafel plots for the various catalysts derived froma. (c) Comparison ofηrequired to initiate HER on various MoS2-only catalysts, including oxygen-incorporated MoS2(ref.26), metallic MoS2(ref.29), superaerophobic MoS2(ref.17), amorphous MoS2(ref.28), defect-rich MoS2(ref.25), MoS2quantum dots18and vertically aligned MoS2film30. (d) Comparison ofηrequired to generate a current density of 10 mA cmgeo−2on various MoS2-based catalysts, including MoS2/N-doped carbon nanotube (CNT)49, Li–MoS2/carbon fibre37, MoS2/graphene33, metallic MoS2(ref.29), defect-rich MoS2(ref.25), amorphous MoS2(ref.28), MoO3/MoS2NWs19and MoS2/CNT-graphene38. (e) EIS Nyquist plots of bulk MoS2and synthesized MoS2nanosheets. Inset shows Nyquist plots at high-frequency range.Z′ is the real impendence andZ″ is the imaginary impedance. (f) Plots showing the extraction of theCdlfor different MoS2electrodes. All the measurements were performed in Ar-saturated 0.5 M H2SO4(pH∼0) and the reported data were iR compensated. Figure 3a compares the current densities achieved within a cathodic potential window for the glassy carbon electrodes modified with different catalysts. The featureless polarization curve for bare glassy carbon guarantees a minimal background. Scanning cathodically reveals that the onset potential of H 2 evolution occurs at approximately −0.10 V versus reversible hydrogen electrode (RHE) for the MoS 2 synthesized at 240 °C, beyond which a sharp increase in catalytic reduction current emerges ( Fig. 3a ). The optimum catalyst loading was determined to be 0.28 mg cm −2 ( Supplementary Fig. 7 ). In contrast, MoS 2 prepared at 190 °C and 260 °C mediate hydrogen evolution at larger overpotential ( η ) of 0.15 and 0.12 V, respectively, while bulk MoS 2 offers negligible H 2 -evolving activity. The superior activity of the MoS 2 synthesized at 240 °C is believed to originate from both its edge-terminated and interlayer-expanded structure. The dependence of the logarithmic current density on η (log j – η ) was plotted to probe the HER kinetics. Figure 3b shows that a sharp increase in current density appeared once the onset potential was reached. The linear relationship of log j and η delivers useful kinetic metrics of above catalysts, namely the Tafel slope. The Tafel slope of 49 mV per decade was measured for the MoS 2 synthesized at 240 °C, which is smaller than those of other catalysts except for the state-of-the-art Pt/C catalyst ( Fig. 3b ). This Tafel slope is comparable to or smaller than that of other MoS 2 -only HER catalysts ( Supplementary Table 1 ) and even many MoS 2 -based hybrid catalysts ( Supplementary Table 2 ) reported in literature, indicating the efficient kinetics of H 2 evolution catalysed by the MoS 2 synthesized at 240 °C. The η required for starting HER on various MoS 2 -only catalysts was compared in Fig. 3c , where ET&IE MoS 2 shows a 20–100 mV decrease in η relative to that of documented MoS 2 . The fast HER kinetics also enabled this ET&IE MoS 2 catalyst to reach a high current density of 10 mA cm −2 at η as low as 0.149 V, outperforming most of the MoS 2 -based HER catalysts ( Fig. 3d , Supplementary Tables 1 and 2 ). Exchange current density ( j 0 ), the most inherent measure of HER activity, was carefully determined to evaluate the quality of ET&IE MoS 2 ( Supplementary Fig. 8 ). The j 0 of 9.62 × 10 −3 mA cm −2 for 240 °C sample surpasses the values of 7.59 × 10 −4 mA cm −2 for 190 °C sample and 2.46 × 10 −3 mA cm −2 for 260 °C sample, as well as the j 0 values reported for MoS 2 -only HER catalysts ( Supplementary Table 1 ). Moreover, the turnover frequency of H 2 molecules evolved per second (s −1 ) for ET&IE MoS 2 was determined to be 1.14 s −1 at η of 200 mV, comparing favourably with the reported MoS 2 -only and even some MoS 2 -based hybrid catalysts ( Supplementary Table 3 and Supplementary Note 1 ). These results highlight the exceptional H 2 -evolving efficiency of this new ET&IE MoS 2 . Figure 3: Electrocatalytic hydrogen evolution of the catalysts. ( a ) Polarization curves for HER on bare glassy carbon electrode and modified glassy carbon electrodes comprising MoS 2 nanosheets synthesized from different temperatures, bulk MoS 2 and a high quality commercial Pt/C catalyst. Catalyst loading is 0.28 mg cm −2 for all samples. Sweep rate: 5 mV s −1 . ( b ) Tafel plots for the various catalysts derived from a . ( c ) Comparison of η required to initiate HER on various MoS 2 -only catalysts, including oxygen-incorporated MoS 2 (ref. 26 ), metallic MoS 2 (ref. 29 ), superaerophobic MoS 2 (ref. 17 ), amorphous MoS 2 (ref. 28 ), defect-rich MoS 2 (ref. 25 ), MoS 2 quantum dots [18] and vertically aligned MoS 2 film [30] . ( d ) Comparison of η required to generate a current density of 10 mA cm geo −2 on various MoS 2 -based catalysts, including MoS 2 /N-doped carbon nanotube (CNT) [49] , Li–MoS 2 /carbon fibre [37] , MoS 2 /graphene [33] , metallic MoS 2 (ref. 29 ), defect-rich MoS 2 (ref. 25 ), amorphous MoS 2 (ref. 28 ), MoO 3 /MoS 2 NWs [19] and MoS 2 /CNT-graphene [38] . ( e ) EIS Nyquist plots of bulk MoS 2 and synthesized MoS 2 nanosheets. Inset shows Nyquist plots at high-frequency range. Z ′ is the real impendence and Z ″ is the imaginary impedance. ( f ) Plots showing the extraction of the C dl for different MoS 2 electrodes. All the measurements were performed in Ar-saturated 0.5 M H 2 SO 4 (pH ∼ 0) and the reported data were iR compensated. Full size image We also applied electrochemical impedance spectroscopy (EIS) technique to provide further insight into the electrode kinetics under HER process (that is, adding a η of 0.2 V). The Nyquist plots ( Fig. 3e and inset) show that ET&IE MoS 2 synthesized at 240 °C has the smallest charge transfer resistance ( R ct ) of only 3.13 Ω, indicating the ultrafast Faradaic process and thus a superior HER kinetics. We attribute this measured small R ct to its synergetic ET&IE structure. The edge-terminated feature can ensure an isotropic electron transport from glassy carbon substrate to MoS 2 edges and significantly decrease the resistance for traversed layers. In addition, the expanded interlayer distance can bring beneficial structural and electronic modulations (which will be discussed below), enabling each MoS 2 layer to resemble more closely to a monolayer structure and a better overall conductivity of our ET&IE MoS 2 . The double-layer capacitance ( C dl ), which is proportional to the effective electrochemically active surface area [27] , [32] , was further measured to probe the advantage of the ET&IE structure ( Fig. 3f ). The observed large C dl of 15.3 mF cm −2 for 240 °C sample indicated its high exposure of active edge sites, comparing favourably with other studied catalysts ( Fig. 3f , Supplementary Fig. 9 ) and thus the improved HER activity. HER performance of the MoS 2 nanostructures synthesized at 240°C for different reaction times was compared and the results are presented in Supplementary Figs 10 and 11 . Material stability of ET&IE MoS 2 The long-term stability of ET&IE MoS 2 and associated ability to continuously catalyse the generation of H 2 was examined using chronoamperometry ( j ∼ t ). This quasi-electrolysis process was conducted at a constant η of 200 mV in 0.5 M H 2 SO 4 ( Fig. 4a ). Remarkably, the H 2 evolution can proceed at a sustained current density of −28 mA cm −2 even over 65 h of continuous operation, suggesting the ultrahigh stability of the ET&IE MoS 2 catalyst. The striking stability was further proved by a long-term cyclic voltammetry cycling test operating in the same electrolyte. 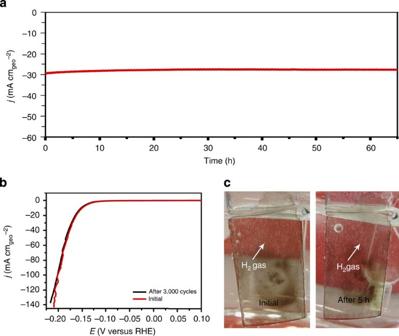Figure 4: HER stability of ET&IE MoS2. (a) Chronoamperometric responses (j∼t) recorded from synthesized ET&IE MoS2at a constant overpotential of 200 mV (no iR compensation). (b) Polarization curves recorded from ET&IE MoS2with a sweep rate of 5 mV s−1before and after 3,000 potential cycles between −0.3 and 0.3 V versus RHE at a sweep rate of 200 mV s−1(with iR compensation). (c) Digital photos show the H2bubbles on ET&IE MoS2-modified FTO before and after 5 h of operation (MoS2loading:∼22.1 μg cm−2). All the measurements were performed in Ar-saturated 0.5 M H2SO4(pH∼0). Figure 4b shows that, after 3,000 cyclic voltammetry cycles, only negligible decay was observed in high current density region, where the massive H 2 bubbles generated at the electrode surface raise the mass transport resistance for the HER. Moreover, this new MoS 2 demonstrates good chemical stability with no obvious degradation of HER activity after storing it under lab environment for 3 months ( Supplementary Fig. 12 ). Digital photos ( Fig. 4c ) taken from the ET&IE MoS 2 -coated fluorine-doped tin oxide (FTO) show vigorous effervescence maintained with no decay even after 5 h of continuous operation while clean FTO is inert ( Supplementary Fig. 13 ). The substantial long-term stability and chemical stability of ET&IE MoS 2 suggest the great promise of using this catalyst to fabricate cost-effective and efficient H 2 evolution electrode in viable water electrolysis systems. Figure 4: HER stability of ET&IE MoS 2 . ( a ) Chronoamperometric responses ( j ∼ t ) recorded from synthesized ET&IE MoS 2 at a constant overpotential of 200 mV (no iR compensation). ( b ) Polarization curves recorded from ET&IE MoS 2 with a sweep rate of 5 mV s −1 before and after 3,000 potential cycles between −0.3 and 0.3 V versus RHE at a sweep rate of 200 mV s −1 (with iR compensation). ( c ) Digital photos show the H 2 bubbles on ET&IE MoS 2 -modified FTO before and after 5 h of operation (MoS 2 loading: ∼ 22.1 μg cm −2 ). All the measurements were performed in Ar-saturated 0.5 M H 2 SO 4 (pH ∼ 0). Full size image HER enhancement mechanism An understanding of intrinsic reasons for the remarkable HER property of ET&IE MoS 2 will be helpful for future HER catalyst design. It is agreed that for a highly active HER catalyst the Gibbs free energy of adsorbed hydrogen (Δ G H ) is close to thermoneutral (that is, Δ G H ≈0) [4] , [23] , [26] . Deviating from this value will make the hydrogen either form a strong bond or not bind efficiently to the catalyst, leading to inefficient hydrogen release and proton–electron transfer and therefore decreased catalytic activity. Recent density functional theory (DFT) calculations revealed that MoS 2 has a Δ G H of 0.08 eV at the Mo edges and should be a good HER catalyst [23] . This prediction was later experimentally verified by the finding that MoS 2 edge sites are highly HER active while its basal planes are inert [24] . Here, our microwave-synthesized MoS 2 preferentially has a high ratio of catalytically active edge sites relative to basal sites due to its highly curved sheet-like structure ( Fig. 2b,e and Supplementary Fig. 1 ), which provides one reason for its striking HER activity. The superior j 0 (9.62 × 10 −3 mA cm −2 ) of the ET&IE MoS 2 relative to that of documented MoS 2 ( Supplementary Table 1 ) prompted us to further consider another underlying enhancement mechanism in this material. Previous reports demonstrated that the electronic structure of MoS 2 can be modified to optimize Δ G H [24] , [26] , [39] , [42] . For example, Co incorporation at S-edges can reduce the Δ G H from 0.18 to 0.1 eV and offer faster proton adsorption kinetics [26] , [39] . Moreover, recent studies have suggested the possibility of engineering the electronic structure of MoS 2 by varying its interlayer distance [29] , [34] , [43] , [44] , [45] , [46] . Kobayashi and Yamauchi reported that a 7% expansion of MoS 2 interlayers is sufficient to render it essentially with a two-dimensional single-layer model [43] . The group of Nørskov performed DFT calculation on the Mo edge of MoS 2 /graphene and found ∼ 0.05 eV change of Δ G H when the interlayer distance has a 0.37 Å discrepancy [46] . To probe the influence of expanded interlayers on their neighbouring couplings, we performed Raman study on ET&IE MoS 2 and compared that with bulk MoS 2 . 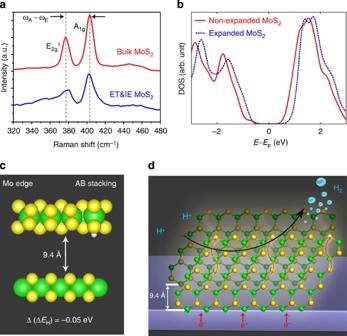Figure 5: HER enhancement mechanism. (a) Raman spectra of bulk MoS2and ET&IE MoS2. (b) The projected DOS on non-expanded MoS2and interlayer-expanded MoS2. (c) DFT calculation of the change in hydrogen adsorption energy (Δ(ΔEH)) between the ET&IE MoS2and non-expanded MoS2. (d) Schematic representation of the edge-terminated MoS2on glassy carbon electrode for HER, where the interlayer spacing is 9.4 Å. Green, yellow and white balls indicate Mo, S and H atoms, respectively. Figure 5a shows that the E 2g 1 mode of ET&IE MoS 2 increases in frequency whereas its A 1g mode exhibits a slight red shift. The smaller separation between the above two modes ( ω A – ω E ) for ET&IE MoS 2 indicates a weakened interlayer mechanical coupling strength, suggesting that ∼ 9.4 Å interlayer gap enables the MoS 2 to approach its single-layer equivalent and thus a modified electronic structure [45] , [47] . Figure 5: HER enhancement mechanism. ( a ) Raman spectra of bulk MoS 2 and ET&IE MoS 2 . ( b ) The projected DOS on non-expanded MoS 2 and interlayer-expanded MoS 2 . ( c ) DFT calculation of the change in hydrogen adsorption energy (Δ(Δ E H )) between the ET&IE MoS 2 and non-expanded MoS 2 . ( d ) Schematic representation of the edge-terminated MoS 2 on glassy carbon electrode for HER, where the interlayer spacing is 9.4 Å. Green, yellow and white balls indicate Mo, S and H atoms, respectively. Full size image We then performed DFT calculations on non-expanded MoS 2 and interlayer-expanded MoS 2 to study the influence of the electronic structure induced by the expanded interlayer distance. Figure 5b shows that the density of states (DOS) of interlayer-expanded MoS 2 is shifted upwards as compared with that of non-expanded MoS 2 , including a shift in the d band of ∼ 0.1 eV towards the Fermi level ( Supplementary Fig. 14 ). This electronic effect will strengthen the H adsorption and offer an increased H coverage on the edge sites [48] . Our calculations also show that the hydrogen adsorption energy (Δ E H ) on Mo edges decreases by about 0.05 eV (a decrease of 0.01 eV on S edges, Supplementary Fig. 15 and Supplementary Note 2 ) for ET&IE MoS 2 as compared to that for non-expanded MoS 2 ( Fig. 5c ). For pristine 2H–MoS 2 , previous calculations revealed that it has a Δ G H of +0.08 eV at the Mo edges with only 25% H coverage under operating conditions and a strengthened H adsorption on the edge sites is needed to improve its activity [23] , [24] . The reduced Δ E H ( ∼ 0.05 eV) of the ET&IE MoS 2 enables an optimized bond strength of the adsorbed H on the Mo edges and thereby a faster proton adsorption kinetics [24] , agreeing well with the DOS results. The advantages of edge-terminated nanostructure that exposes an abundance of active edge sites, as well as the enlarged interlayer distance with modified edge electronic structures, together lead to the high HER performance of this single MoS 2 catalyst ( Fig. 5d ). In summary, we demonstrate a new nanostructured MoS 2 catalyst with edge-terminated and interlayer-expanded features that was synthesized through a microwave heating strategy. The measured HER activity and stability of this MoS 2 structure exceed almost all the documented counterpart MoS 2 and enable the promise for exploring it as a realistic H 2 evolution electrode. Beside the edge-terminated structure that allows more active edge sites, the expanded interlayer distance can further optimize its electronic structure and therefore permits the performance gains. Our results here raise a new catalyst design concept regarding to layered materials through modulating their interlayer coupling. Material synthesis All chemicals were used as received without further purification. In a typical synthesis, 10 mg (NH 4 ) 2 MoS 4 (99.97%, Sigma-Aldrich) was added to 6 ml DMF (anhydrous, 99.8%, Sigma-Aldrich) followed by stirring for 15 min under ambient condition. The resulting solution was transferred into a 10 ml microwave reaction vessel, which was then heated to 240 °C at the fast ramp and the temperature was maintained for 2 h in a microwave reactor (CEM corporation) operated under the sealed vessel mode. The reaction solution was cooled to room temperature with pressurized nitrogen flow and the resulting black product was collected via centrifugation (8,000 r.p.m. for 5 min). The precipitate was washed with distilled water and absolute ethanol for at least four times to remove ions and possible remnants, followed by drying at 60 °C in an oven for 4 h. For the time-dependent experiment, the temperature was set at 240 °C while reactions stopped at different times; for the temperature-dependent experiment, the reaction time was 2 h while the reaction temperatures were altered intentionally, all the corresponding products were collected for further studies. Characterization The as-synthesized samples were examined by X-ray powder diffraction was carried out on a Bruker D2 Phaser X-ray diffractometer with Cu Ka radiation ( λ =1.5406 Å) at 30 kV and a current of 10 mA. The morphology of the as-synthesized samples was determined by using a JEOL 2010F(s) TEM. The HRTEM observation and SAED were taken on the same machine with an acceleration voltage of 200 kV. The energy-dispersive X-ray spectra were collected with an INCA X-ray microanalysis system equipped on the JEOL 2010F(s) microscope. All samples were prepared by dropping the ethanol suspension containing uniformly dispersed nanocrystals onto the carbon-coated copper grids and dried at room temperature naturally. Raman spectra were performed using a Raman microscope (Renishaw) excited with a 514 nm excitation laser. The Fourier transform infrared (FTIR) spectra were measured on a Thermo Fisher/Nicolet 6,700 FTIR spectrometer at room temperature. Electrocatalytic study Electrochemical measurements were performed at room temperature using a rotating disk working electrode made of glassy carbon (PINE, 5 mm diameter, 0.196 cm 2 ) controlled by a CH Instruments 700C potentiostat. The glassy carbon electrode was polished to a mirror finish and thoroughly cleaned before use. Pt coil and double junction Ag/AgCl (PINE, 4 M KCl) were used as counter and reference electrodes, respectively. All the potentials reported in this work were normalized against that of the RHE. The preparation method of the working electrodes containing investigated catalysts can be found as follows. In short, 5 mg of catalyst powder was dispersed in 1 ml of 3:1 vol/vol deionzed water/isopropanol mixed solvent, which was ultrasonicated for about 30 min to generate a homogeneous ink (no Nafion solution was added due to the ink can form intact and stable film on glassy carbon electrode). Then, 10 μl of the dispersion was transferred onto the glassy carbon disk, leading to the catalyst loading of 0.28 mg cm −2 . Finally, the as-prepared catalyst film was dried at room temperature. For comparison, bare glassy carbon electrode that has been polished and cleaned was also dried for electrochemical measurement. Before the electrochemical measurement, the electrolyte (0.5 M H 2 SO 4 ) was degassed by bubbling pure argon for at least 0.5 h to ensure the saturation of the electrolyte. The polarization curves were obtained by sweeping the potential from −0.35 to 0.15 V versus RHE at room temperature and 1,600 r.p.m (to remove the in situ formed H 2 bubbles on the RDE), with a sweep rate of 5 mV s −1 . The electrochemical impedance spectroscopy measurement was performed in the same configuration at overpotential of 200 mV over a frequency range from 5 MHz to 5 mHz at the amplitude of the sinusoidal voltage of 5 mV and room temperature. The MoS 2 synthesized at 240 °C for 2 h was spin coated onto FTO-coated glass slide (Sigma-Aldrich, surface resistivity ∼ 7 Ω per square; 1.5 cm × 2.5 cm; catalyst loading 22.1 μg cm −2 ) and used as working electrode to perform chronoamperometry experiments at various overpotentials. Cyclic voltammograms performed at various sweep rates were used to estimate the C dl were recorded in the potential region of 0.1–0.2 versus RHE at room temperature. The polarization curves were replotted as overpotential ( η ) versus log current (log j ) to get Tafel plots for assessing the HER kinetics of investigated catalysts. By fitting the linear portion of the Tafel plots to the Tafel equation ( η = b log ( j ) + a ), the Tafel slope ( b ) can be obtained. DFT calculations The hydrogen adsorption energy (Δ E H ) calculations on strip models of non-expanded MoS 2 and ET&IE MoS 2 were performed by periodic DFT using the plane wave code Vienna Ab-initio Simulation Package (VASP). The change in hydrogen adsorption energies is reported as Δ(Δ E H ). Structural models are represented using the visualization tool Visualization for Electronic and STructural Analysis (VESTA). Details of the calculation and relevant references are provided in the Supplementary Note 3 . How to cite this article: Gao, M.-R. et al. Edge-terminated molybdenum disulfide with a 9.4-Å interlayer spacing for electrochemical hydrogen production. Nat. Commun. 6:7493 doi: 10.1038/ncomms8493 (2015).